Nanoelectromechanical coupling in fullerene peapods probed by resonant electrical transport experiments Fullerene peapods, which are carbon nanotubes encapsulating fullerene molecules, can offer enhanced functionality with respect to empty nanotubes. Their prospective applications include, for example, data storage devices, single-electron transistors and spin-qubit arrays for quantum computing. However, the present incomplete understanding of how a nanotube is affected by entrapped fullerenes is an obstacle for peapods to reach their full potential in nanoscale electronic applications. In this paper, we investigate the effect of C 60 fullerenes on low-temperature electron transport through peapod quantum dots. Compared with empty nanotubes, we find an abnormal temperature dependence of Coulomb blockade oscillations, indicating the presence of a nanoelectromechanical coupling between electronic states of the nanotube and mechanical vibrations of fullerenes. This provides a method to detect the C 60 presence and to probe the interplay between electrical and mechanical excitations in peapods, which thus emerge as a new class of nanoelectromechanical systems. Since their discovery [1] , single wall carbon nanotubes (SWNTs) encapsulating arrays of C 60 fullerene molecules [2] , [3] , the so-called fullerene peapods, have attracted a lot of interest among physicists, chemists, as well as among materials and electrical engineers. Peapods are considered as potential building blocks in nanoelectronics, offering enhanced functionality with respect to empty nanotubes. Their prospective applications include data storage devices [4] , single-electron transistors [5] , [6] , [7] , [8] and spin-qubit arrays for quantum computing [9] . Nevertheless, the extent to which the electronic properties of peapods, critical for their applications, are affected by entrapped fullerenes is still unclear. Theoretical studies [10] , [11] , [12] predict dramatic changes in the electronic band structure of the nanotube, because of hybridization and corresponding shifts of SWNT energy states and C 60 molecular orbitals. This was supported by scanning tunnelling microscopy experiments [13] and photoluminescence excitation/emission mapping [14] . On the other hand, no fundamental perturbation of the nanotube electron system was found in photoemission experiments [15] and in electrical transport measurements on peapods [6] , [7] , [8] . In the latter case, quantum effects dominated device characteristics at low temperatures in the same manner as for empty nanotubes: clean electron transport with signatures of Kondo physics [16] was observed through peapods functioning as single or double quantum dots (QDs) in the regime of strong electronic coupling Γ between energy states of the dot and its electrical leads. Coherent transport was also found for peapods filled with Sc@C 82 metallofullerenes [17] , the incorporation of which, in principle, should have an even stronger effect on the nanotube's band structure than C 60 molecules. In this paper, we study the effect of the encapsulated C 60 fullerenes on low-temperature electron transport through peapod QDs in the regime of weak electronic coupling. Compared with empty nanotubes, we find an abnormal temperature dependence of Coulomb blockade [18] (CB) conductance oscillations, indicating a modification of single-electron excitations at low temperatures. These novel elementary excitations, which appear as a result of C 60 encapsulation, can be explained by a nanoelectromechanical coupling between quantized electronic states of the nanotube and the mechanical vibrations of fullerenes. Their appearance provides a method to detect the C 60 presence and to probe the interplay between electrical and mechanical degrees of freedom in fullerene peapods, which emerge as a new class of nanoelectromechanical systems (NEMS). We stress that other types of devices for which a coupling to mechanical vibrations plays a crucial role in electrical transport are molecular conductors [19] and transistors [20] , as well as suspended nanotubes [21] , [22] . 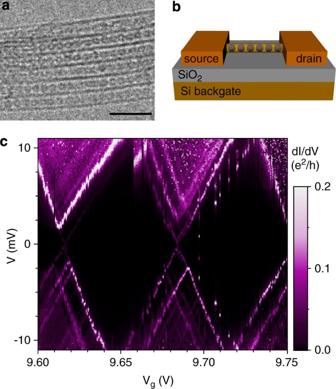Figure 1: C60fullerene peapod device. (a) Transmission electron microscopy image of C60peapods with densely packed fullerene chains. The scale bar is 5 nm. (b) Schematic layout of the device. An individual C60peapod deposited on a SiO2substrate is contacted by Pd/Au source and drain electrodes, spaced 400 nm apart. (c) Stability diagram of a C60peapod. Colour-coded differential conductance dI/dVis measured atT=0.3 K as a function of backgate voltageVgand bias voltageV, showing the diamond-shaped features characteristic of the Coulomb blockade. Fullerene peapod devices Figure 1a shows a transmission electron microscopy image of our peapod material, containing SWNTs densely filled with C 60 molecules. For electrical transport measurements, individual peapods with a diameter of 1.3–2 nm were contacted by Pd/Au source and drain electrodes, as schematically illustrated in Fig. 1b . (See Methods for more details on devices.) The C 60 peapods showed clear CB behaviour at low temperatures ( Fig. 1c ), indicating that single-electron charging effects dominated the low-temperature electrical transport. Both the charging energy U ≈8–12 meV and the electronic level spacing Δ E ≈2–3 meV corresponded well to a 400-nm-wide separation between contact electrodes, suggesting that individual peapod QDs were defined by tunnel barriers at the peapod–electrode interfaces. Because QDs were probed at gate voltage ranges corresponding to a reduced electronic coupling Γ to the leads, no zero-bias Kondo anomaly [6] , [7] was observed here. Figure 1: C 60 fullerene peapod device. ( a ) Transmission electron microscopy image of C 60 peapods with densely packed fullerene chains. The scale bar is 5 nm. ( b ) Schematic layout of the device. An individual C 60 peapod deposited on a SiO 2 substrate is contacted by Pd/Au source and drain electrodes, spaced 400 nm apart. ( c ) Stability diagram of a C 60 peapod. Colour-coded differential conductance d I /d V is measured at T =0.3 K as a function of backgate voltage V g and bias voltage V , showing the diamond-shaped features characteristic of the Coulomb blockade. 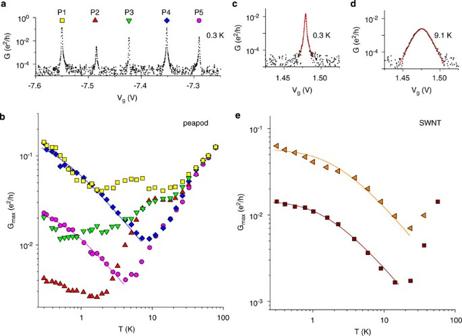Figure 2: Temperature dependence of linear conductance. (a) CB oscillations in the linear conductanceG=dI=dV|V=0, measured as a function of gate voltageVgfor a C60fullerene peapod. (b) Maximal conductance amplitudeGmaxversus temperatureT, determined for the five peaks indicated in (a). Peaks P4 and P5 behave as predicted by the Breit–Wigner (BW) model, whereas others show an abnormal temperature dependence. (c) and (d) Lineshape of a conductance peak for a reference SWNT device, measured at 0.3 K and 9.1 K, respectively. These lineshapes correspond to a thermally broadened Breit–Wigner peak. At low temperatures,kBT≪Γ, the peak approaches the Lorentzian lineshapeGBW(E)∝1/[(E–E0)2+(Γ/2)2], as apparent in (c). At higher temperatures,kBT≫Γ, it can be approximated by a negative derivative of the Fermi function,G(E)∝-∂f/∂E, see (d). (e)GmaxversusTfor the reference SWNT device. As predicted by the BW theory,Gmax(T) is nearly independent ofTat low temperatures,kBT≪Γ, whereas at higher temperatures,kBT≫Γ, the 1/Tbehaviour is clearly recovered. In (b–e), the thin solid lines indicate fits to the experimental data performed using the Breit–Wigner model. Full size image CB oscillations Figure 2a depicts the linear conductance G of a fullerene peapod as a function of gate voltage V g , revealing CB oscillations. As CB peaks appear when an energy state in the QD lines up with the Fermi level of the leads, this kind of experiment is a basic tool for probing both the energy spectrum and wavefunctions of elementary excitations in a QD: the positions of the peaks provide information about the spectrum, whereas the magnitude of the tunnelling current is proportional to the overlap between the wavefunctions of the incident electron and the elementary excitation in the dot. The temperature dependence of the heights of the five CB peaks that appear in Fig. 2a is shown in Fig. 2b . Figure 2: Temperature dependence of linear conductance. ( a ) CB oscillations in the linear conductance G =d I =d V | V =0 , measured as a function of gate voltage V g for a C 60 fullerene peapod. ( b ) Maximal conductance amplitude G max versus temperature T , determined for the five peaks indicated in ( a ). Peaks P4 and P5 behave as predicted by the Breit–Wigner (BW) model, whereas others show an abnormal temperature dependence. ( c ) and ( d ) Lineshape of a conductance peak for a reference SWNT device, measured at 0.3 K and 9.1 K, respectively. These lineshapes correspond to a thermally broadened Breit–Wigner peak . At low temperatures, k B T ≪ Γ, the peak approaches the Lorentzian lineshape G BW (E) ∝ 1/[( E – E 0 ) 2 +(Γ/2) 2 ], as apparent in ( c ). At higher temperatures, k B T ≫ Γ, it can be approximated by a negative derivative of the Fermi function, G (E) ∝ -∂f/∂ E , see ( d ). ( e ) G max versus T for the reference SWNT device. As predicted by the BW theory, G max ( T ) is nearly independent of T at low temperatures, k B T ≪ Γ, whereas at higher temperatures, k B T ≫ Γ, the 1/ T behaviour is clearly recovered. In ( b–e ), the thin solid lines indicate fits to the experimental data performed using the Breit–Wigner model. Full size image The lineshape and temperature response of CB oscillations in the linear conductance have been widely investigated in the past [18] , [23] , both for metal and semiconductor QDs. In the CB regime in which electron transport occurs only through a single electronic dot level, the tunnelling probability as a function of energy is given by the Breit–Wigner formula (see caption to Fig. 2 ). The temperature dependence of conductance peaks is therefore entirely due to thermal broadening of the energy of the incident electrons: The peak height G max is independent of temperature T in the low-temperature limit, where k B T ≪ Γ. Here, k B is the Boltzmann's constant, and k B T the thermal energy. In the opposite high-temperature limit, k B T ≫ Γ, a universal 1/ T -behaviour is observed. This corresponds to what we observed for empty SWNTs, as shown in Figs 2c–e . For fullerene peapods, however, the measured temperature dependence of conductance peaks is often significantly different (see Fig. 2b ), implying that the Breit–Wigner picture is no longer valid. We interpret this discrepancy as a signature of a change in the spectrum of the elementary excitations and of their wavefunctions, a change that can be associated with encapsulated fullerenes. 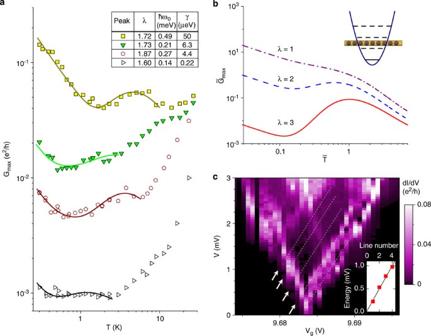Figure 3: Polaronic interactions in a fullerene peapod. (a)GmaxversusTfor conductance peaks with an abnormal temperature behaviour with respect to the Breit–Wigner model. Solid and open symbols indicate data points measured for two different peapod devices. Solid lines are fits to the experimental data calculated using the polaronic model described in the text. The inset gathers the determined fitting parameters. (b, inset) A schematic diagram of the harmonic potential defining the oscillating motion of the vibrator, with horizontal lines representing vibronic energy states spaced byℏω0. At temperatureskBT≪ℏω0, only the ground state (solid line) participates in the conductance. As soon askBTbecomes of the order ofℏω0, thermally excited vibronic modes are generated (dashed lines). (b, main figure) Calculated renormalized peak conductancevs reduced temperaturefor three values of the electron–vibron coupling λ. At low temperatures,kBT≪ℏω0, an exponential suppression of the conductance occurs,, because of a reduced overlap between the electronic wavefunction in the lead and the polaronic wavefunction in the dot. Here, is the thermally broadened BW peak conductance for non-interacting electrons. The stronger the polaronic coupling λ, the stronger the suppression of the conductance. By increasing the temperature, the competition between thermally generated vibrons and polarons gives rise to a non-monotonic behaviour. An abnormal temperature dependence of the peak height is particularly well visible forkBT≫λ2ℏω0where conductance is dominated by the term. At higher temperatures,kBT≫λ2ℏω0, the polaronic blockade is completely overcome by thermal excitations and the conductance scales as 1/T, following the Breit–Wigner formula. See Methods for more details on the model. (c) A closer look at a stability diagram dI=dVversusVversusVg. Arrows and thin dashed lines indicate weak quasi-periodic excitation lines running parallel to the Coulomb diamond edge. The inset shows their excitation energies; the solid line has a slope of 0.25 meV. Typically, as highlighted in Figure 3a , an anomalous temperature dependence is observed on the scale of a few kelvin. The corresponding energy is of the order of 0.1 meV, which is small on the electronic energy scale but relevant for the longitudinal vibrational motion of the encapsulated fullerenes. (For the low-diameter peapods used in our study, the characteristic scale of transverse vibrations would be ∼ 1 meV.) Figure 3: Polaronic interactions in a fullerene peapod. ( a ) G max versus T for conductance peaks with an abnormal temperature behaviour with respect to the Breit–Wigner model. Solid and open symbols indicate data points measured for two different peapod devices. Solid lines are fits to the experimental data calculated using the polaronic model described in the text. The inset gathers the determined fitting parameters. ( b , inset) A schematic diagram of the harmonic potential defining the oscillating motion of the vibrator, with horizontal lines representing vibronic energy states spaced by ℏ ω 0 . At temperatures k B T ≪ ℏ ω 0 , only the ground state (solid line) participates in the conductance. As soon as k B T becomes of the order of ℏ ω 0 , thermally excited vibronic modes are generated (dashed lines). ( b , main figure) Calculated renormalized peak conductance vs reduced temperature for three values of the electron–vibron coupling λ. At low temperatures, k B T ≪ ℏ ω 0 , an exponential suppression of the conductance occurs, , because of a reduced overlap between the electronic wavefunction in the lead and the polaronic wavefunction in the dot. Here, is the thermally broadened BW peak conductance for non-interacting electrons. The stronger the polaronic coupling λ, the stronger the suppression of the conductance. By increasing the temperature, the competition between thermally generated vibrons and polarons gives rise to a non-monotonic behaviour. An abnormal temperature dependence of the peak height is particularly well visible for k B T ≫ λ 2 ℏ ω 0 where conductance is dominated by the term . At higher temperatures, k B T ≫ λ 2 ℏ ω 0 , the polaronic blockade is completely overcome by thermal excitations and the conductance scales as 1/ T , following the Breit–Wigner formula. See Methods for more details on the model. ( c ) A closer look at a stability diagram d I =d V versus V versus V g . Arrows and thin dashed lines indicate weak quasi-periodic excitation lines running parallel to the Coulomb diamond edge. The inset shows their excitation energies; the solid line has a slope of 0.25 meV. Full size image Nanoelectromechanical coupling To interpret our experimental results, we use a model in which SWNT electrons are electromechanically coupled to a set of low-frequency vibrators: single C 60 fullerenes [24] or their clusters, trapped by a longitudinal harmonic potential inside the nanotube. Within this approach, the peapod is treated as a multilevel QD for which each quantized electronic level is selectively coupled to a single vibrational mode, in a manner similar to that in the local Holstein model [25] , and the corresponding dimensionless electron–vibron coupling constant λ is proportional to the amplitude of vibronic quantum fluctuations. As a result, the resonant tunnelling electrons can be dressed by vibrational excitations if they spend sufficiently long time in the dot to form real electron–vibron hybrids—Holstein polarons [24] . As the probability of polaron formation is enhanced for long electron dwell times in the QD, τ ∝ 1/Γ, polaronic effects become more pronounced in the regime of weak electronic coupling Γ. We stress that electron–vibron coupling does not have any significant effect on the fullerene vibrations themselves, as they are mostly determined by the C 60 confinement within the carbon nanotube. Even though the coupling to each electronic level may be strong and depend on the position of the oscillating fullerenes, their total energy shift averages out over a large number of individual electronic states in the dot. Our model calculations ( Fig. 3b ) have revealed qualitatively similar features to those experimentally observed for conductance peaks deviating from conventional Breit–Wigner behaviour ( Fig. 3a ). In particular, three characteristic thermal regimes can be distinguished: (1) When the thermal energy is much smaller than the vibration energy, k B T ≪ ℏ ω 0 , conductance is suppressed for strong electron–vibron coupling λ l. (Here, ℏ is the reduced Planck's constant and ω 0 is the angular frequency of vibrations.) Such a polaronic (or Franck-Condon) blockade of conductance [26] signals the reduced probability for an electron to tunnel from a pure electronic state in the lead to a polaronic state in the dot, and vice versa. (2) As the temperature rises, the population of the thermally excited vibronic levels increases, following the Bose distribution n ( z ) with z= ℏ ω 0 / k B T . This has a destructive effect on the polaronic wavefunction, leading to a non-monotonic behaviour of conductance in the temperature interval k B T λ 2 ℏ ω 0 , where λ 2 ℏ ω 0 represents the characteristic energy of a polaron. (3) At high temperatures, k B T ≫ λ 2 ℏ ω 0 , polaronic effects are lifted and conductance takes the standard Breit–Wigner form, G max ∝ 1/ T . To determine the electron–vibron coupling λ in the peapod devices, we have numerically fitted the temperature dependence of conductance maxima ( Fig. 3a ) with the thermal progression predicted by our model (equation (5) in Methods). The obtained fits are in good agreement with the experimental data, yielding large values for the polaronic coupling parameter, λ =1.6–1.9. These values are consistent with the suppression of the conductance observed at low temperatures. They are also of the same order of magnitude as in previous experiments on suspended carbon nanotube devices [21] , [22] , in which vibronic states were due to intrinsic modes of the SWNT. (Note that in study by Sapmaz et al . [21] and Leturcq et al . [22] , the coupling constant was defined as g = λ 2 .) The inset to Fig. 3a gathers all the fitting parameters extracted for the investigated peaks. The vibrational origin of the abnormal features observed in G max ( T ) is in addition supported by the appearance of weak, quasi-periodic excitation lines along the edges of CB diamonds in the stability diagrams, as indicated by arrows in Fig. 3c . The mean energy spacing ∼ 0.25 meV of these nearly equidistant excitations is an order of magnitude smaller than the electronic level spacing Δ E =2–3 meV in our 400-nm-long peapod QDs. On the other hand, it closely matches the values of vibrational quanta extracted from the fits to G max ( T ), see the inset to Fig. 3a . Our experimental data clearly indicate that not all of the studied conductance peaks show abnormal features in their temperature dependence, see Fig. 2b . This observation can be explained if, for different SWNT electron states n , there are strong fluctuations [24] in the value of the polaronic coupling constant. Such fluctuations may be due to a local character of the nanoelectromechanical coupling. Consequently, only for some electronic levels is the characteristic time needed to form a polaronic state ℏ /( λ n 2 ℏ ω 0 ) sufficiently shorter than the electron dwell time in the dot ℏ /Γ n . We note here that electronic coupling Γ could not be directly determined from the polaronic fits. Instead, we were able to probe a related parameter γ =Γ L Γ R /(Γ L +Γ R ), yielding γ =0.004–0.050 meV, for the investigated conductance peaks. Here, Γ L and Γ R are electronic couplings to the left and right reservoir of the QD, respectively, and Γ=Γ L +Γ R . Assuming symmetrical barriers, Γ L =Γ R , the value of Γ could thus be evaluated as Γ=4 γ . For the asymmetric coupling, Γ L =10 Γ R , this would yield Γ=12.1 γ . To gain an insight into the nature of the vibrational motion of fullerene molecules trapped inside a SWNT, we have performed a simple estimation of the potential that confines their longitudinal oscillations. The confining potential can be readily obtained from Girifalco's universal potential for graphitic structures [27] if we assume that it is mainly due to the interaction of a vibrating C 60 molecule with its nearest neighbour molecules (one on each side). The resulting potential is well approximated by a harmonic potential characterized by force constant k =2.2 Nm −1 . The corresponding vibrational energy quantum ℏ ω 0 matches the value of about 0.25 meV, which is needed to fit the experiments, for a particle mass that is about 10 times larger than that of a single C 60 molecule ( ). The implication is that the relevant molecular vibrations may involve clusters of about 10 C 60 molecules. (Within this estimation, a cluster is considered to be a group of neighbour molecules vibrating in phase.) For peapods with densely packed fullerene chains, clusters of this size could form inside the SWNT, for example, as a result of local tube corrugations or due to the presence of defects (openings) on the SWNT side wall [2] . Such deformations would locally alter van der Waals forces defining the average distance [27] between fullerenes and the nanotube and between neighbouring fullerenes, thus leading to a redistribution of C 60 molecules to minimize the potential energy. The incomplete understanding of how a nanotube is affected by encapsulated fullerenes is an obstacle for peapods to reach their full potential in nanoelectronic applications. [4] , [5] , [6] , [7] , [8] , [9] The experiments presented here shed light on this issue. They demonstrate the presence of nanoelectromechanical coupling in carbon peapods, which thus emerge as a new class of NEMS. Moreover, the characterization technique described here can be thought of as a tool for detecting the presence of fullerenes, or other molecules, in a nanotube. Such an experimental verification can be performed in situ for individual tubes in electronic devices, unlike in other detection techniques that require either a large ensemble of peapods (Raman spectroscopy [28] , X-ray diffraction [29] ) or probing in dedicated systems (transmission electron microscopy, scanning tunnelling microscopy [13] , low-temperature atomic force microscopy [30] ). Further studies using suspended peapods could allow a tuning of the fullerenes' spatial distribution within the nanotube by means of mechanical bending deformations of the SWNT. If the resonant character of electron transmission could be controlled mechanically by these means or by others, carbon peapods could find applications as NEMS resonators, with an operation frequency set by the vibrational motion of the encapsulated fullerenes in the 100 GHz range. Devices The high-quality fullerene peapods investigated in our study were based on arc discharge-grown SWNTs. The empty tubes (also used as reference SWNTs) were supplied by NANOCARBLAB as a purified material (80% pure grade). Because of the purification procedure (multi-step heating in air, soaking in HNO 3 , microfiltration), the as-received SWNTs were already opened and required no further treatment before being filled with C 60 fullerenes (98% purity, INTERCHIM). Filling was carried out by the vapour phase method [2] in an evacuated and sealed ampoule at 500 °C for 24 h. To remove excess fullerenes, heat treatment was performed later under dynamic vacuum at 800 °C for 1 h. Transmission electron microscopy indicated that 90–95% of the tubes in the resulting material encapsulated fullerenes (that is, were peapods). A quantitative analysis by X-ray diffraction [29] confirmed that the peapods were densely packed with C 60 molecules, with a filling ratio of ∼ 80%. In addition, signatures of the encapsulated C 60 fullerenes were found in Raman spectroscopy. The peapods (or the reference empty nanotubes) were sonicated in dichloroethane and deposited on a silicon wafer covered with silicon oxide. Individual tubes with a diameter of 1.3–2 nm were located and selected for further processing by means of atomic force microscopy. Electron beam lithography was then used to define the source and drain electrodes of Pd/Au (15 nm/45 nm), with a spacing of 400 nm. A highly n-doped Si substrate, situated beneath the 500-nm-thick SiO 2 layer, served as a backgate. Electrical transport experiments were performed in a 3 He cryostat with a base temperature of T =300 mK. Model We highlight here the main steps of our theoretical modelling, which is based on the local Holstein model [25] . More details can be found in the study by Krive et al . [24] To obtain analytical results, we assume that only one vibrating scatterer (a cluster of fullerenes or a single molecule) is confined inside the SWNT. The full Hamiltonian for a two-terminal peapod QD system reads as follows: where is the Hamiltonian for the Fermi leads and α = L,R for the left and right reservoir, respectively. The peapod-QD Hamiltonian reads as follows: where { ɛ n } is the set of energy levels in the dot, ℏ ω 0 is the vibrational quantum of energy, , L is the length of the dot, x=l is the position of the scatterer, ν F is the Fermi velocity of SWNT electrons, and x 0 is the amplitude of the zero-point fluctuations of the bosonic field. c n ( c n † ) and b ( b † ) are fermionic and bosonic operators with canonical commutation relations. The longitudinal motion of the scatterer in the SWNT is defined by a harmonic potential. Finally, the tunnelling Hamiltonian reads as follows: where we assume that the hopping matrix elements t between the two leads and the dot are of the same order. The above QD Hamiltonian can be diagonalized by a unitary transformation, which reveals that the major effect of the vibrational bosonic field is to renormalize the energy levels in the dot. These levels are shifted by an amount λ n 2 ℏ ω 0 , the so-called polaronic shift, where is the electron–vibron coupling constant. To obtain the expression for the conductance of our system, we start from the Meir–Wingreen formula [31] where f L/R ( ɛ ) are the Fermi functions for the left and right reservoirs, γ =Γ L Γ R /(Γ L +Γ R ); Γ L/R =2 πt 2 ρ L/R are the widths of the resonance due to tunnelling from the left or right lead, and ρ L/R are the densities of states in the reservoirs. G QD ret ( ɛ ) is the retarded Green function of the dot that can be evaluated in the wide-band limit [32] . By means of gate voltage, an energy level in the QD can be tuned to line up with the Fermi level ɛ F in the leads, so that ɛ F = ɛ n – λ n 2 ℏ ω 0 . This is when the conductance reaches its maximum. In the linear conductance regime, one finds that the temperature dependence of these maxima is given by the simple expression where is the standard resonance conductance of a single-level QD. In equation 5, the function F λ ( z ), with z = ℏ ω 0 / k B T , can be expressed as a series, where I l is the modified Bessel function of the first kind and n ( z ) is the Bose distribution function. The thin solid lines in Fig 3a show fits to the experimental data obtained with the help of expression 5 for the conductance. How to cite this article: Utko, P. et al . Nanoelectromechanical coupling in fullerene peapods probed by resonant electrical transport experiments. Nat. Commun. 1:37 doi: 10.1038/ncomms1034 (2010).